Nitrogen cycle feedbacks as a control on euxinia in the mid-Proterozoic ocean Geochemical evidence invokes anoxic deep oceans until the terminal Neoproterozoic ~0.55 Ma, despite oxygenation of Earth’s atmosphere nearly 2 Gyr earlier. Marine sediments from the intervening period suggest predominantly ferruginous (anoxic Fe(II)-rich) waters, interspersed with euxinia (anoxic H 2 S-rich conditions) along productive continental margins. Today, sustained biotic H 2 S production requires NO 3 − depletion because denitrifiers outcompete sulphate reducers. Thus, euxinia is rare, only occurring concurrently with (steady state) organic carbon availability when N 2 -fixers dominate the production in the photic zone. Here we use a simple box model of a generic Proterozoic coastal upwelling zone to show how these feedbacks caused the mid-Proterozoic ocean to exhibit a spatial/temporal separation between two states: photic zone NO 3 − with denitrification in lower anoxic waters, and N 2 -fixation-driven production overlying euxinia. Interchange between these states likely explains the varying H 2 S concentration implied by existing data, which persisted until the Neoproterozoic oxygenation event gave rise to modern marine biogeochemistry. Enrichments in reactive iron are a consistent feature of marine sediments throughout most of the Proterozoic [1] , [2] , [3] , [4] , indicating persistent ocean anoxia well after Earth’s first major rise in atmospheric oxygen (the Great Oxidation Event) at ~2.32 Ga (ref. 11 ). The emerging picture now suggests a predominance of ferruginous conditions in the deep ocean [1] , [2] , [3] , with euxinic conditions along productive continental shelves and in epicontinental seas, likely having a key role in reducing Fe(II) concentrations in comparison to before the Great Oxidation Event [6] ( Fig. 1 ). The contrast between expanded euxinia during the Proterozoic and the rarity of sulphidic conditions today [7] , [8] suggests that the two periods experienced a different balance of marine biogeochemical feedbacks. It is particularly intriguing that euxinic conditions recurred at the Precambrian–Cambrian boundary [9] and in association with subsequent ocean anoxic events (OAEs), with potential relevance to mass extinctions [10] . Interestingly, some such OAEs appear on the basis of isotopic and biomarker evidence to have coincided with high rates of nitrogen fixation in the surface ocean [11] . A related link between Proterozoic euxinia and nitrogen cycle perturbation via trace element stress has been suggested [12] , but quantitative support for this ‘bioinorganic bridge’ hypothesis is presently lacking [13] . 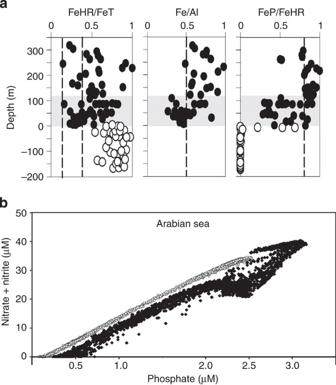Figure 1: Contemporary evidence implies that the significant euxinia observed in the ancient ocean involved a disturbance in Redfield N:P stoichiometry. (a) Proterozoic geochemical data suggest sulphidic conditions that were sufficiently abundant and widespread to leave a geochemical signature, and modern oceanographic data suggest that such conditions may involve a link to the nitrogen cycle—we argue here that these two observations are connected. Upper figure shows an example geochemical profile of Fe data from Proterozoic continental margin sediments from 1.88–1.83 Ga (ref.3). Open circles represent iron formation, filled circles indicate siliciclastics. A high reactive fraction of total FeHR: Fetotal> 0.38 suggests anoxic conditions (left), high Fe relative to Al (middle) supports the notion of Fe enrichment (because this measure is unaffected by subsequent removal of reactive Fe(II) species). The pyritized fraction of reactive iron (right), distinguishes euxinic Fepyr: Fe > 0.8 from ferruginous Fepyr: FeHR< 0.8 conditions. Geochemical profiles from the Proterozoic ocean frequently suggest a ferruginous deep ocean with euxinic incursions at intermediate depths on continental margins. (b) Assuming that sulphidic conditions equate to a loss of nitrate, data from the (rare) modern coastal upwelling zones in which NO3−is exhausted before PO43−suggests that a link to nitrogen fixation may be relevant (lower graph, see discussion in8). Black diamonds show anoxic water columns influenced by N2production, open circles show adjacent water bodies unaffected by anoxic conditions. Note the greater relative excess of phosphate relative to nitrate in the former. Figure 1: Contemporary evidence implies that the significant euxinia observed in the ancient ocean involved a disturbance in Redfield N:P stoichiometry. ( a ) Proterozoic geochemical data suggest sulphidic conditions that were sufficiently abundant and widespread to leave a geochemical signature, and modern oceanographic data suggest that such conditions may involve a link to the nitrogen cycle—we argue here that these two observations are connected. Upper figure shows an example geochemical profile of Fe data from Proterozoic continental margin sediments from 1.88–1.83 Ga (ref. 3 ). Open circles represent iron formation, filled circles indicate siliciclastics. A high reactive fraction of total Fe HR : Fe total > 0.38 suggests anoxic conditions (left), high Fe relative to Al (middle) supports the notion of Fe enrichment (because this measure is unaffected by subsequent removal of reactive Fe(II) species). The pyritized fraction of reactive iron (right), distinguishes euxinic Fe pyr : Fe > 0.8 from ferruginous Fe pyr : Fe HR < 0.8 conditions. Geochemical profiles from the Proterozoic ocean frequently suggest a ferruginous deep ocean with euxinic incursions at intermediate depths on continental margins. ( b ) Assuming that sulphidic conditions equate to a loss of nitrate, data from the (rare) modern coastal upwelling zones in which NO 3 − is exhausted before PO 4 3− suggests that a link to nitrogen fixation may be relevant (lower graph, see discussion in [8] ). Black diamonds show anoxic water columns influenced by N 2 production, open circles show adjacent water bodies unaffected by anoxic conditions. Note the greater relative excess of phosphate relative to nitrate in the former. Full size image Denitrification yields substantially more free energy per mole of organic carbon oxidized than dissimilatory sulphate reduction (−398 kJ mol −1 compared with −43.8 kJ mol −1 (ref. 14 )), meaning that denitrification will be the dominant anaerobic respiratory pathway when both electron acceptors are bioavailable. This competitive exclusion on energetic grounds may be part of the reason why sustained sulphidic conditions are rare even in modern oxygen minimum zones [8] . These basic observations suggest that the most problematic aspect of explaining euxinia that was sufficiently sustained/widespread to leave a geochemical signature in the rock record is envisaging a situation in which there is simultaneously minimal denitrification and appreciable organic carbon available for sulphate reducers. Exhausting nitrate may initially seem a plausible explanation, but the fact that NO 3 − is a limiting nutrient causes a self-limiting negative feedback that reduces the supply of organic matter to be respired—unless there is some alternative source of fixed nitrogen to the surface ocean [8] , [15] , [16] . Today, nitrate can only become exhausted in conjunction with significant new production when that production is supported by N 2 fixation. This is responsible for the (rare) sulphide build-up that occasionally occurs during coastal upwelling events [7] , [8] , [16] . Here we explore the implications of these simple feedbacks in the context of the Proterozoic ocean, specifically in terms of the ongoing discussion [17] , [18] about what caused significant euxinia to occur against the backdrop of largely ferruginous conditions. We use a simple five-box model [8] of a coastal upwelling zone ( Fig. 2 ), in which we resolve export production and the apportioning of its respiration between various potential electron acceptors (full model description given in the Supplementary Methods and in the original paper by Canfield [8] ). We focus on the nutrient composition and mass balance of the upwelling zone, into which newly fixed organic carbon sinks from the photic zone, and is subsequently respired in a manner dictated by electron-acceptor availability, according to the hierarchy in free energy yield O 2 >NO 3 − >SO 4 2− . (In the context of the minimalist approach taken here, we neglect Fe(III) respiration, primarily because it is difficult to envisage any unambiguous difference in its magnitude between the N 2 fixation and non-fixation cases on which we focus). Based on a mass balance for the concentration of limiting nutrient upwelling into the photic zone, we obtain an estimate of new production, which dictates the export production available for heterotrophic respiration in the lower water column. We derive organic carbon respiration fluxes that are consistent with simultaneous steady-state organic carbon and electron acceptor concentrations (see Methods and Table 1 ). 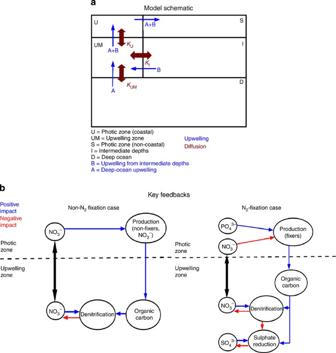Figure 2: A minimalistic feedback-based model. Model schematic (a) and summary of key feedbacks (b) operating in the presence and absence of nitrogen fixation. The upper diagram shows the five-box model we use (ref.8). We focus on nutrient composition and biogeochemical fluxes in the upwelling zone UM, which is driven by export production from the photic zone U, and nutrient upwelling from the deep D and intermediate depth I regions. Nutrient concentrations are buffered by mixing with non-coastal surface S and intermediate depth I boxes. The results we show below constitute an analysis of the sensitivity that the upwelling zone’s nutrient composition has to the rate of advective upwelling from intermediate depths B (including the other advective upwelling parameter A in the analysis does not qualitatively alter the results). In the feedback diagram, blue arrows denote a positive influence, red arrows denote a negative influence. A circular feedback loop that contains an even number of red arrows constitutes a net positive-feedback loop, one that contains an odd number of red arrows constitutes a net negative-feedback loop. Black arrows denote physical mixing (diffusion and/or upwelling). The key difference between the fixation case (b, right) and non-fixation case (b, left) is that in that in the latter case NO3−acts simultaneously as a limiting nutrient in the photic zone and (under anoxic conditions) a respiratory electron acceptor in the upwelling zone. This means that increasing denitrification causes a net negative feedback on (NO3−-limited) export production, preventing nitrate exhaustion. In the fixation case, the rate of new production is not subject to this feedback. Figure 2: A minimalistic feedback-based model. Model schematic ( a ) and summary of key feedbacks ( b ) operating in the presence and absence of nitrogen fixation. The upper diagram shows the five-box model we use (ref. 8 ). We focus on nutrient composition and biogeochemical fluxes in the upwelling zone UM, which is driven by export production from the photic zone U, and nutrient upwelling from the deep D and intermediate depth I regions. Nutrient concentrations are buffered by mixing with non-coastal surface S and intermediate depth I boxes. The results we show below constitute an analysis of the sensitivity that the upwelling zone’s nutrient composition has to the rate of advective upwelling from intermediate depths B (including the other advective upwelling parameter A in the analysis does not qualitatively alter the results). In the feedback diagram, blue arrows denote a positive influence, red arrows denote a negative influence. A circular feedback loop that contains an even number of red arrows constitutes a net positive-feedback loop, one that contains an odd number of red arrows constitutes a net negative-feedback loop. Black arrows denote physical mixing (diffusion and/or upwelling). The key difference between the fixation case ( b , right) and non-fixation case ( b , left) is that in that in the latter case NO 3 − acts simultaneously as a limiting nutrient in the photic zone and (under anoxic conditions) a respiratory electron acceptor in the upwelling zone. This means that increasing denitrification causes a net negative feedback on (NO 3 − -limited) export production, preventing nitrate exhaustion. In the fixation case, the rate of new production is not subject to this feedback. Full size image Table 1 Summary of solutions used in different contexts. Full size table In contrast to the implementation of the model for a modern oxygenated ocean by Canfield [8] (also see Supplementary Fig. S1 ), we include the explicit possibility of electron-acceptor limitation of denitrification, and separate new production into components based on reductive assimilation of NO 3 − and on direct assimilation of NH 4 + . Our results constitute a ‘snapshot’ of a simple, chemically continuous coastal upwelling region in a context representative of the Proterozoic ocean. We provide a simple analysis of the sensitivity that the nutrient composition of this region has to the presence or absence of nitrogen fixation, in each case relative to changes in upwelling rate. Our objective is to determine the circumstances in which euxinia can be sustained in a way that is consistent with local steady-state nutrient composition (rather than to quantitatively resolve global biogeochemical budgets). Model parameters are given in the Supplementary Table S1 , broadly representative of surface ocean oxygen levels equating to ~0.1 present atmospheric level (see Supplementary Figures S2–S4 for a sensitivity analysis), with an anoxic, [19] , [20] Fe(II) rich, [1] , [2] deep ocean assumed as the default state. Dissociation between NO 3 -driven production and euxinia The key result is that H 2 S can build-up at intermediate depth when nitrogen fixation supports production at the surface ( Fig. 3b ), but not when nitrogen fixation is absent ( Fig. 3a ). Changes in the rate of upwelling from the deep ocean quantitatively alter export production fluxes and respiration rates, but the association between N 2 fixation and H 2 S build-up is, as in the modern system [8] , [16] a robust result. (Because fixers will be outcompeted by non-fixers where NO 3 − is available, we only consider model results from the nitrogen-fixation case when photic zone nitrate is lower in concentration than the value required for Redfield stoichiometry with phosphate). We include the nitrification of aerobically remineralized organic nitrogen (anaerobically remineralized organic nitrogen is assumed to remain as NH 4 + ), which acts as an input of NO 3 − to the upwelling waters, and (via eddy diffusion) to the photic zone. Consequently, oxic conditions below the photic zone can, by regenerating and oxidizing organic nitrogen, cause NO 3 − concentration to rise in the photic zone, meaning that the occurrence of nitrogen fixation is no longer plausible as a steady state. A thorough analysis of the sensitivity that the results have to the oxygen concentration in the boxes surrounding the upwelling zone is shown in Supplementary Figs S2–S4 . Naturally, the assumed baseline oxygen concentration has a quantitative impact on the fluxes - but does not alter the basic distinction between the feedbacks operating in the fixation and non-fixation cases. 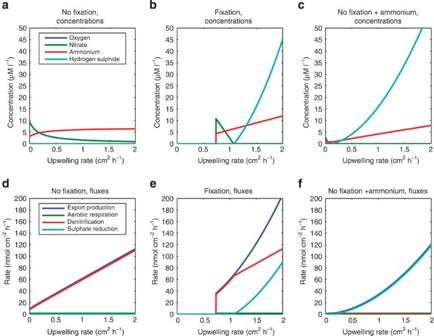Figure 3: The impact of the nitrogen-fixation state on the occurrence of sulphidic conditions. Nutrient concentrations (a–c) and biogeochemical fluxes (d–f) in the upwelling zone for non-fixation (a,d), fixation (b,e) and non-fixation/ammonium (c,f) cases referred to in the main text. Concentration of ferrous iron, oxygen representative of an incompletely oxygenated upper ocean at 0.1 PAL and an anoxic deep ocean,, nitrate set to roughly modern values ocean,, sulphate concentrations set to 0.1 present day(raising sulphate levels does not alter the results because sulphate reduction is carbon limited), and phosphate concentrationsrepresentative of a low productivity ocean without the modern terrestrial weathering input. In the non-fixation case (a,d), the negative feedback between nitrate and production prevents sulphide build-up. In the fixation case (b,e), the constraint that nitrate must be below Redfield stoichiometry with phosphate confines the steady state results to the high-production, anaerobic region of parameter space, within which sulphide build-up occurs as soon as nitrate is exhausted. The absence of nitrate in the ammonium case (c,f) means that sulphide build-up occurs as soon as the upwelling zone goes anoxic. The qualitative distinction between the three states on which we focus is not sensitive to parameter choices. A sensitivity analysis to the prescribed ammonium and oxygen concentrations in the boxes surrounding the upwelling zone is shown in theSupplementary Information, but does not qualitatively alter the results. Figure 3: The impact of the nitrogen-fixation state on the occurrence of sulphidic conditions. Nutrient concentrations ( a – c ) and biogeochemical fluxes ( d – f ) in the upwelling zone for non-fixation ( a , d ), fixation ( b , e ) and non-fixation/ammonium ( c , f ) cases referred to in the main text. Concentration of ferrous iron , oxygen representative of an incompletely oxygenated upper ocean at 0.1 PAL and an anoxic deep ocean , , nitrate set to roughly modern values ocean , , sulphate concentrations set to 0.1 present day (raising sulphate levels does not alter the results because sulphate reduction is carbon limited), and phosphate concentrations representative of a low productivity ocean without the modern terrestrial weathering input. In the non-fixation case ( a , d ), the negative feedback between nitrate and production prevents sulphide build-up. In the fixation case ( b , e ), the constraint that nitrate must be below Redfield stoichiometry with phosphate confines the steady state results to the high-production, anaerobic region of parameter space, within which sulphide build-up occurs as soon as nitrate is exhausted. The absence of nitrate in the ammonium case ( c , f ) means that sulphide build-up occurs as soon as the upwelling zone goes anoxic. The qualitative distinction between the three states on which we focus is not sensitive to parameter choices. A sensitivity analysis to the prescribed ammonium and oxygen concentrations in the boxes surrounding the upwelling zone is shown in the Supplementary Information , but does not qualitatively alter the results. Full size image Deep-ocean ammonium as a key uncertainty If an ammonium source additional to that derived from anaerobic remineralization is assumed to exist at steady state in the deep ocean and upwell into the photic zone, non-fixation-driven production is decoupled from the negative feedback with nitrate. Such a scenario can therefore, in theory, give rise to euxinia in the absence of N 2 fixation, subject to this clause of a significant deep-ocean ammonium source ( Fig. 3c , also see additional results with higher prescribed deep/intermediate ocean ammonium concentrations given in Supplementary Figs S5–S7 ). High ammonium scenarios are arguably representative of a reversion to an Archaean-like reduced nitrogen cycle [21] , in which the NO 3 − -based component of the modern nitrogen cycle is assumed to be less significant, because low oxygen availability limits nitrification. Such a scenario may be plausible, particularly further back into the early Proterozoic. Indeed, it is worth mentioning in this context that it has been quantitatively argued that the ancient nitrogen cycle itself may have created an oxygen sink that significantly contributed to the delay between atmospheric and ocean oxygenation—because the initial build-up of a nitrate pool requires that the system pass through a ‘bottleneck’ in which oxygen consumption during nitrification and (after nitrate-driven export production) denitrification of organic matter exceeds oxygen production by nitrate-assimilation-driven primary production [22] . All these arguments are consistent with the results of our simple model, and would dictate the interchange between the three states shown in Fig. 3 , as well as the oxygen/ammonium boundary conditions involved ( Supplementary Information ). However, our purpose here is to propose a consistent explanation for the occurrence of euxinia in the mid-late Proterozoic, based on the initial assumption of an oxygenated photic zone. With this in mind it is difficult to view the ammonium case ( Fig. 2c ) as a long-term steady state, because an ammonium pool upwelling into the photic zone would undergo nitrification immediately below the depth to which light penetrated. Nitrification can occur in industrial biofilm reactors down to O 2 concentrations of ~30 μM (ref. 23 ), and isotopic evidence has been interpreted as indicating an onset of nitrification and associated ‘oxic’ nitrogen cycle processes as early as 2.67 Ga (ref. 24 ). Given these arguments, and indeed as the evidence for ocean oxygenation is pushed back into the Neoproterozoic [25] , it becomes less likely that an upwelling ammonium pool could support export production without leading to concurrent build-up of nitrate (therefore denitrification, therefore a lack of sulphate reduction). The ammonium case is therefore probably a transient scenario that separates the fixation and non-fixation cases. Predicted anticorrelation between δ 15 N and euxinia A possible test of the notion of nitrogen cycle control on Proterozoic/Neoproterozoic euxinia could be found in a comparison between δ 15 N and Fe pyritization ( Fig.4a ). We hypothesize that Proterozoic data sets (when considered as an ensemble) should exhibit evidence for an association between nitrogen fixation in the photic zone and euxinia in the lower anoxic water column, and (in the non-fixation case) for an association between denitrification and non-euxinic conditions. Specific predictions include (for example) that biomarker/isotopic evidence for nitrogen fixation should be systematically associated with the Fe pyritization diagnostic of euxinia in the mid/late Proterozoic—exactly as observed in Cretaceous OAEs [10] , [26] . Equivalently, there should be a systematic anticorrelation between any denitrification signature (for example, positive δ 15 N of kerogen equilibrated with water column nitrate) and evidence for euxinia. We illustrate the latter prediction in Fig. 4a by coupling our steady-state model results to a semiquantitative estimate of nitrate δ 15 N, comprising fractionations from assimilatory nitrate reduction, nitrification and denitrification (but neglecting fixation). The δ 15 N of kerogen in sediments is assumed to reflect the isotopic composition of the nitrate with which the organic matter was in contact [27] —thus a water column influenced by high rates of denitrification will produce kerogen with a positive ( 15 N-enriched) δ 15 N signal. A crucial prediction of the N-cycle feedback control that we hypothesize here is that if any such positive δ 15 N signal diagnostic of denitrification is found after a systematic examination of Proterozoic sediments, it will be decoupled in time and space from the pyritization of reactive Fe. 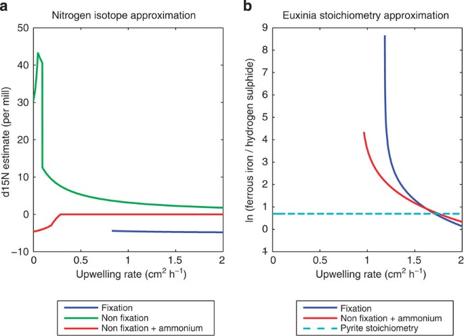Figure 4: Example testable predictions from the feedback-based hypothesis that we suggest. Left graph (a) shows an approximate estimate of the δ15N signature of water column NO3−(per mil) incorporating the15N/14N fractionations from nitrification, nitrate assimilation and water column denitrification, for the fixation (blue), non-fixation (green) and non-fixation with NH4+(red) upwelling cases. In the fixation case, the signal is dominated by nitrification of remineralized ammonium, and (low) nitrate assimilation (note that results for upwelling rate less thanB=0.8 are disregarded because they result in nitrate concentration being too high to permit fixers to occur). In the ammonium/non-fixation case, there is a nitrification signal until the upwelling zone goes anoxic, from which point the signal is neutral due to the absence of any nitrate. In the non-fixation, nitrate case, there is a strong positive signal from water column denitrification, which is dampened as nitrate concentration declines and is subsequently dominated by the other two fractionations. The right hand graph (b) shows the natural logarithm of the upwelling zone Fe(II)/H2S ratio (for those cases in which sulphide is produced—the fixation (blue) and non-fixation ammonium-driven (red) scenarios). Note that any set of parameter choices giving rise to a positive δ15N signal is inconsistent with sufficient sulphide availability to permit FeS2precipitation. The impact of ammonium assimilation on nitrate δ15N is discussed in theSupplementary Information, and although this and other fractionations may make interpretation of a δ15N signal more complex, it will not affect the separation in upwelling parameter space between genuine denitrification and euxinia signatures that we argue for. Figure 4: Example testable predictions from the feedback-based hypothesis that we suggest. Left graph ( a ) shows an approximate estimate of the δ 15 N signature of water column NO 3 − (per mil) incorporating the 15 N/ 14 N fractionations from nitrification, nitrate assimilation and water column denitrification, for the fixation (blue), non-fixation (green) and non-fixation with NH 4 + (red) upwelling cases. In the fixation case, the signal is dominated by nitrification of remineralized ammonium, and (low) nitrate assimilation (note that results for upwelling rate less than B =0.8 are disregarded because they result in nitrate concentration being too high to permit fixers to occur). In the ammonium/non-fixation case, there is a nitrification signal until the upwelling zone goes anoxic, from which point the signal is neutral due to the absence of any nitrate. In the non-fixation, nitrate case, there is a strong positive signal from water column denitrification, which is dampened as nitrate concentration declines and is subsequently dominated by the other two fractionations. The right hand graph ( b ) shows the natural logarithm of the upwelling zone Fe(II)/H 2 S ratio (for those cases in which sulphide is produced—the fixation (blue) and non-fixation ammonium-driven (red) scenarios). Note that any set of parameter choices giving rise to a positive δ 15 N signal is inconsistent with sufficient sulphide availability to permit FeS 2 precipitation. The impact of ammonium assimilation on nitrate δ 15 N is discussed in the Supplementary Information , and although this and other fractionations may make interpretation of a δ 15 N signal more complex, it will not affect the separation in upwelling parameter space between genuine denitrification and euxinia signatures that we argue for. Full size image In addition to an estimate of nitrate δ 15 N, we include the model upwelling zone’s Fe(II)/H 2 S concentration relative to the threshold value of 2 stoichiometrically consistent with pyrite formation ( Fig. 4b ). Steady-state iron concentration was dictated by the concentration upwelling from the deep ocean, parameter choices of which were intended to be representative of ferruginous conditions [19] , [20] . The key point is that the signatures for denitrification and for euxinia always occur in different regions of parameter space—a separation that should be reflected in the real record by a sustained, widespread and ultimately qualitative separation between the fixation/euxinic and non-fixation/ferruginous cases. Our nitrogen isotope estimate is intended only as a rough approximation and an example of the type of data cross-referencing exercise that could be conducted for the Proterozoic (when appropriate data become available) to improve understanding of marine biogeochemical evolution in a testable way. We focus on the processes that distinguish the presence and absence of euxinia, rather than attempt to build a comprehensive nitrogen isotope model. One process that we neglect in the main results for simplicity, but that could conceivably be relevant to the δ 15 N signal is ammonium assimilation—an analysis of the effect of which we include in Supplementary Figs S8–S11 . For example, if an ammonium pool becomes 15 N-enriched due to preferential (but non-quantitative) assimilation of the lighter isotope, and then this water column ammonium is subsequently nitrified, this will increase the δ 15 N of the resultant nitrate. Conversely, if the source of ammonium for nitrification is anaerobically remineralized organic nitrogen, the δ 15 N of the nitrate that results will be decreased. The quantitative balance between ammonium assimilation and remineralization, and various other fractionations within the wider Proterozoic nitrogen cycle are near-impossible to constrain in any systematic way that can be related to the presence/absence of euxinia. Although such processes might make it difficult to unambiguously identify a denitrification-specific δ 15 N signal, they do not alter the basic result that any genuine denitrification signal will not occupy the same region of parameter space as Fe pyritization and other evidence for euxinia. The Fe(II) concentration of real Proterozoic upwelling zones was likely influenced by the balance between heterotrophic respiration using Fe 3+ as an electron-acceptor and chemo-litho-autotrophic oxidation of Fe 2+ in conjunction with nitrate reduction [14] . In some contexts an association between Fe(II) oxidation and nitrate reduction may even have made ferruginous and nitrate-rich conditions incompatible at steady state, perhaps ultimately leading to ammonium production, net loss of bioavailable nitrogen via anammox and a switch back to the fixation case. Anammox itself is likely highly relevant to the wider Proterozoic nitrogen budget and the transition between the fixation and non-fixation cases, and anaerobic ammonium oxidation coupled to Fe(III) reduction might logically be expected to be substantial at the interface between an oxygenated photic zone and a ferruginous deep ocean. However, as a chemoautotrophic process, anammox is unlikely to be of crucial relevance to the apportioning between respiratory electron acceptors, and in general it is again difficult to envisage a predictable way in which any of these (important) processes would influence the nitrogen cycle–euxinia link. Our results and steady-state approach is intended to apply to a typical coastal upwelling region within the mid-late Proterozoic ocean. We work subject to the starting assumptions (i) that the photic zone/upper water column was well-oxygenated and (ii) that the existing evidence for a relative abundance of highly reactive iron, an appreciable fraction of which intermittently became pyritized, is genuinely representative of typical continental margins within the global ocean, and changes in the average biogeochemical composition of the upwelling regions in those areas. Clearly it is also entirely reasonable to envisage a situation within which bodies of water with the distinct nutrient compositions we have referred to are simply separated in space (but not time) within the same ocean. Nevertheless, the basic biogeochemical feedbacks that must have operated in the ancient ocean as today dictate that one of the limiting cases, in Fig. 2 , must still have applied. Relaxing our simplistic steady-state approach, for example, by using a dynamical, spatially explicit representation of bodies of water with distinct nutrient compositions would require constraints on the circulation patterns/internal structure of the Proterozoic ocean that are (at present) near-impossible to obtain. The modelling philosophy we have adopted here is that, as for most deep time problems, given the uncertainties in the magnitudes of the fluxes it is preferable to focus on the feedbacks and use simple models as a device for making testable predictions. Our simple model is sufficient to show that the feedbacks, which today confine sulphidic conditions to very rare contexts, also imply that changes in the nitrogen cycle dictated changes in euxinia during the Proterozoic. Although changes in water column stratification and/or global sulphate budgets [28] are, of course, relevant to euxinia, we argue that the ‘electron tower’ of respiratory-free energy yield [14] dictates that nitrate availability is a stronger first-order control. Similarly, the ongoing debate as to the significance of trace element limitation leading to stalls at various points in the nitrogen cycle [12] , [13] , [29] , [30] is not theoretically inconsistent with our arguments and may yet gain empirical validation. We suggest that as data become more available the empirical community should conduct a systematic cross-referencing exercise between the implicit occurrence of euxinia and the presence/absence of nitrogen fixation/nitrate-limited production. Speaking in terms of global averages and geological timescales, if euxinia was widespread and persistent, bioavailable nitrate and the processes dependent on them must have been equivalently scarce. The Precambrian–Cambrian boundary therefore marks not only ocean oxygenation, but a fundamental change in the feedbacks that sustained the primary production. The ultimate cause of the interchange between the fixation and non-fixation cases was presumably dictated, as today, by the occurrence (or not) of a nitrate deficit relative to Redfield stoichiometry with phosphate [31] , which constrains the nutrient composition of all primary producers in the ocean, and means that only nitrogen fixers can grow when such a deficit occurs [31] , [32] . Phosphate input from weathering is an obvious candidate driver for periods of nitrogen fixation (therefore euxinia) during the Proterozoic, one which could conceivably have been enhanced (above the previous non-biologically enhanced rate) by colonization of the land surface [37] towards the end of the Neoproterozoic. In a similar speculative vein, the basic idea that sulphate-reducing bacteria spent an appreciable fraction of their evolutionary past in an environment experiencing bioavailable nitrogen stress is circumstantially supported by the observation that sulphate reducers are capable of facultative nitrogen fixation [33] . It is even conceivable that nitrogen fixation under euxinic conditions could produce a negative δ 15 N signature [34] which future geochemical data may record, and which would work in the same direction as our semiquantitative isotopic predictions. If our arguments are correct, it would imply that global productivity occurred in the context of two distinct N-cycle states, fixation/euxinic and non-fixation/non-euxinic, between which an interchange occurred in time and/or space until the Neoproterozoic oxygenation event caused anoxic conditions to become a much more localized/transient phenomenon, permitting the sustainable build of a nitrate pool and making nitrogen fixation itself a more spatially contextual phenomenon. The end of the Proterozoic would thereby constitute the origin of the modern ‘nitrostat’ [31] , [32] , giving rise to the feedbacks that sustain habitability in the modern ocean. A simple model of upwelling zone respiratory fluxes Canfield’s [8] five-box model (see Fig. 2 and Supplementary Fig. S1 ) resolves the apportioning of respiration of export production among electron acceptors in an upwelling zone, linked by diffusion to photic zone, deep and intermediate depth boxes. Vertical diffusion occurs over a length scale of 20–100 m, horizontal diffusion over 100 km 1 (ref. 10 ). The magnitude of the export production flux sinking into the upwelling zone scales stoichiometrically with limiting nutrient concentration in the photic zone (nitrate in the non-fixation case, phosphate in the fixation case). The basic approach is to solve for limiting nutrient concentration in the photic zone, use this to estimate export production from the photic zone to the upwelling zone, solve for each steady-state electron acceptor concentration in the upwelling zone and work out (stoichiometrically) what fraction of export production respiration this electron-acceptor concentration implies—assuming electron acceptor preferential use in the order O 2 >NO 3 − >SO 4 2− due to free energy yield differences (for example, [35] , [36] , please note the free energy yields below are per mole of reaction, not per mole organic carbon as referred to in the main text and reference 14): The original model was modified so as to be applicable to a Proterozoic ocean by (i) separating export production into components based on assimilatory nitrate reduction and direct ammonium assimilation, (ii) explicitly including the potential for electron-acceptor limitation of denitrification and (iii) inclusion of Fe parameters and coupling to a semiquantitative nitrate δ 15 N estimate. The nutrient composition of the upwelling zone follows from writing a simple steady-state mass balance for oxygen O 2 , phosphate P, sulphate S, reactive ferrous iron Fe R and bioavailable nitrogen—subdivided into oxidized N ox and reduced N R ‘pools’. Organic carbon fluxes comprise export production EP, aerobic respiration R aerobic , denitrification R denif and sulphate reduction R SR . We focus on the respired (that is, non-buried) fraction of photic zone export production, which we equate to the sum of aerobic respiration, denitrification and sulphate reduction EP= R aerobic + R denif + R SR , the relative magnitude of which depends, of course, on electron-acceptor availability. Where sulphide build-up occurs, it scales stoichiometrically with the sulphate reduction flux. To understand the following derivations the reader is asked to refer to Fig. 2 (and Canfield [8] ), and to keep in mind the following abbreviations. The five boxes are the coastal photic zone U, the non-coastal surface ocean S, the coastal upwelling zone UM, the non-coastal intermediate depth ocean I and the deep ocean D. A given flux is simply the product of the concentration of the relevant nutrient in the box and some mixing parameter—either diffusive (K j for box j) or via advective upwelling (A and B). Non-N 2 -fixation case Lack of N 2 fixation in the photic zone implies bioavailable nitrate is at or in excess of Redfield stoichiometry to phosphate and therefore that NO 3 − and/or NH 4 + feeds directly into photic zone (suffix U) production by non-N 2 -fixing photoautotrophs. The export production flux thus scales with upwelling of bioavailable nitrogen into the photic zone: Oxic upwelling zone When the upwelling zone remains oxic, all export production is consumed by aerobic respiration R aerobic =EP. Writing an oxygen mass balance: (Where the various ‘r’ coefficients above and below are stoichiometric conversion parameters, see Supplementary information ). We assume that all aerobically respired organic nitrogen is nitrified after remineralization, so feeds into the nitrate N ox pool, whereas anaerobic remineralization of organic nitrogen adds to the ammonium pool N R . The mass balance for reduced nitrogen is: The mass balance for oxidized nitrogen is: For the oxic case all respiration is aerobic R total = R aerobic =EP (note we neglect organic carbon burial here in order to avoid introducing an unnecessary free parameter, so export production is equal to total remineralization in the upwelling zone), so we get reduced nitrogen concentration directly from (3): Where bioavailable photic zone ammonium (and nitrate) is zero for steady state, because it feeds straight into a new production. Substituting (5) into (1), then (1) into (4) (recalling that R aerobic =EP), then solving for nitrate: We now know oxygen by (2), (5), (6) and R total = R aerobic =EP: Anoxic upwelling zone If (7) does not give a non-zero estimate for upwelling zone oxygen concentration, then we assume that respiration of export production drives the upwelling zone anoxic at steady state. We approximate the aerobic respiration flux that sustains anoxic conditions at steady state by using (7) with : We now need to apportion the remaining carbon available for anaerobic respiration between denitrification and sulphate reduction. Carbon-limited denitrification If there is sufficient nitrate in the upwelling zone to oxidize all remaining carbon (that is, if denitrification is carbon-limited not electron-acceptor-limited), then we write an organic carbon mass balance using (1): Then, rewriting the nitrate mass balance (4) to include both the input from nitrification of aerobically remineralized organic nitrogen and the output from denitrification, we have: Inserting (9) into (10) and solving for nitrate: The remaining unknown is ammonium. Inserting (9) and then (11) into (3), (recalling that at steady state because nitrogen is the limiting nutrient) then rearranging and solving for ammonium concentration: Nitrate-limited denitrification If the estimate of nitrate concentration that we arrive at from (11) is less than or equal to zero, we assume that there is insufficient nitrate to oxidize all the organic carbon available for anaerobic respiration and that we therefore need a different way in which to determine the denitrification flux that sustains the nitrate-limited steady state, which we can then use to calculate sulphate reduction. (Note that the inclusion of this potential scenario in the non-fixation case illustrates how the absence of sulphate reduction associated with it is a genuine model output, because the theoretical potential for sulphate reduction without nitrogen fixation is built into the model). It is here that the separation of new production into components based on nitrate and ammonium assimilation is useful, because it prevents the system being underdetermined. First, we rewrite the organic carbon mass balance for in (1), insert this into (3) retaining for steady state because nitrogen is limiting, then solve for upwelling zone ammonium: As discussed above, nitrate is a limiting nutrient and cannot be exhausted at the same time as supporting sufficient production to drive its exhaustion by denitrification. To formalize this, we write a separate carbon balance for the nitrate-fuelled component of export production , and we equate this to the electron-acceptor-limited denitrification flux: We then rewrite (10) but with in the water column and insert (14) instead of RdenifClimited. That is, we substitute in the nitrate-limited denitrification flux and solve for the nitrate concentration going through that flux when NO 3 − =0 at steady state in the water column. Equation (15) simply shows that for nitrate concentration to limit the rate of denitrification at the same time as supporting export production from higher up in the water column, there must be a significant reserve of nitrate coming in from deep/intermediate depth regions of the ocean and/or nitrification of aerobically remineralized organic nitrogen must still be possible. Export production is now fully constrained for nitrate-limited denitrification, and the actual denitrification flux consistent with this is: We can now finally write a carbon balance to estimate the rate of sulphate reduction in the electron-acceptor-limited denitrification, non-nitrogen-fixation case substituting (15) and (16) into the organic carbon balance: In other words, sulphate reduction necessarily scales with upwelling zone ammonium concentration. Photic zone nitrogen fixation Non-zero nitrogen fixation necessarily requires a lack of bioavailable nitrate in the photic zone (else N 2 -fixers will be outcompeted due to the energetic cost of the process). Consequently, we impose a stoichiometry criterion: Unless inequality (18) is true (that is, unless there is a bioavailable nitrogen deficit in comparison to Redfield stoichiometry with phosphate) we set export production to zero for the fixation case. When this is realized, export production scales with phosphate upwelling into the photic zone: Writing a phosphate mass balance for the upwelling zone: The steady-state phosphate concentration comes from inserting (19) into (20): Once again we need to determine whether there is sufficient oxygen to remineralize all export production, or whether the upwelling zone goes anoxic. Rewriting (2) with EP= R aerobic , inserting (21) into (19) and writing a mass balance for oxygen: Oxic upwelling zone If (22) gives a non-zero estimate for upwelling zone oxygen concentration, then we get nitrate concentration straight away from (4): Anoxic upwelling zone If (22) does not permit non-zero oxygen then we assume aerobic respiration is again given by (8), and we rewrite the nitrate mass balance (10), replacing the denitrification term with : If (24) gives a non-zero nitrate concentration, then we assume (as above) that denitrification consumes all the organic carbon available after aerobic respiration. However, such a significant nitrate pool is, of course, unrealistic at steady state in the fixation case. If denitrification does occur in the fixation case we assume that it exhausts any residual nitrate, so is the minimum of the solution of (10) for and the left over carbon However, in practice, denitrification is close to zero for all the fixation case results. The remaining organic carbon feeds into sulphate reduction, which we get by substituting in (25), (21), (19) and (8) into a final organic carbon mass balance: In each of the results discussed in the main text, the ratio of reactive iron to sulphate comes from a mass balance for the (parameterized) iron concentrations, related to the sulphide output from sulphate reduction: Additional equations, a fully referenced list of parameter choices, and an explanation of the nitrogen isotope approximation are given in the Supplementary Information . How to cite this article: Boyle, R.A. et al . Nitrogen cycle feedbacks as a control on euxinia in the mid-Proterozoic ocean. Nat. Commun. 4:1533 doi: 10.1038/ncomms2511 (2013).